Monogamy and haplodiploidy act in synergy to promote the evolution of eusociality In eusocial species, some individuals sacrifice their own reproduction for the benefit of others. The evolutionary transition towards eusociality may have been facilitated by ancestral species having a monogamous mating system (the monogamy hypothesis) or a haplodiploid genetic system (the haplodiploidy hypothesis), or it may have been entirely driven by other (ecological) factors. Here we show, using a model that describes the dynamics of insect colony foundation, growth and death, that monogamy and haplodiploidy facilitate the evolution of eusociality in a novel, mutually reinforcing way. Our findings support the recently questioned importance of relatedness for the evolution of eusociality, and simultaneously highlight the importance of explicitly accounting for the ecological rules of colony foundation, growth and death in models of social evolution. Eusocial insects show a degree of organization and integration at the colony level that has earned them the label of 'super-organisms' [1] . The transition from a solitary lifestyle to eusociality poses a problem for the Darwinian [2] account of evolution by natural selection, because it requires the evolution of altruistic traits that contradict the principle of individual fitness maximization [3] . A general solution to this problem was outlined by Hamilton's insight that, despite the principle of 'survival of the fittest', the ultimate criterion that determines whether a gene G for an altruistic behaviour will spread 'is not whether the behaviour is to the benefit of the behaver but whether it is to the benefit of the gene G ...' [4] . However, the biological mechanisms by which this principle manifests itself during evolutionary transitions are still incompletely understood. The idea that haplodiploidy can facilitate this transition has suffered a decline [5] , [6] , [7] , recent data suggest a greater role for monogamy [8] , [9] , and a lively debate has ensued around the role kin selection has in the process [7] , [10] , [11] , [12] . To show that haplodiploidy and monogamy can work synergistically to promote eusociality when demographic and genetic rules of colony growth are properly accounted for, here we envisaged a species whose genetic system is either haplodiploid or diplodiploid, and in which females mate with either one (monandry) or with two males (biandry) before beginning to reproduce. Male offspring always disperse from the nest, whereas female offspring exhibit one of two phenotypes: a reproductive phenotype that disperses and seeks to reproduce, and a 'worker' phenotype that stays with the mother as a non-reproductive helper. We let the probability of developing each phenotype be determined by a diploid locus with a 'solitary' (dispersive) and a 'eusocial' allele. A queen's reproductive rate b ( n ) increases as a function of colony size n (with a parameter s defining the 'returns to scale' which determine how much more efficiently larger colonies convert resources into offspring; we assume either increasing or decreasing returns to scale, Fig. 1 ). For simplicity, once a colony has reached its maximum size N , newly produced offspring disperse by default. Our findings add further to the understanding of eusociality. 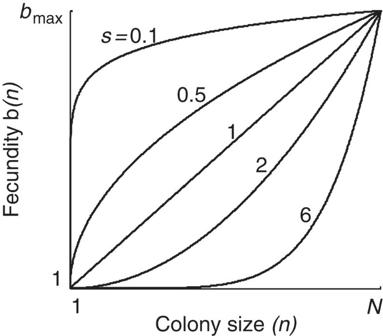Figure 1: Female fecundity as a function of colony size. The function is given byb(n)=1+(bmax−1)*((n−1)/(N−1))s. The 'returns to scale' are constant with shape parameters=1 and increasing ifs>1. Figure 1: Female fecundity as a function of colony size. The function is given by b ( n )=1+( b max −1)*(( n −1)/( N −1)) s . The 'returns to scale' are constant with shape parameter s =1 and increasing if s >1. Full size image Evolutionary dynamics The dynamics of our model exhibits areas of parameter space where the frequency of the eusocial allele increases or decreases from given ancestral states ( Figs 2 , 3 , 4 , 5 ): a eusocial area, where the eusocial allele spreads to fixation from any starting frequency; a mixed area, where either allele spreads if rare, leading to stable polymorphism (coexistence of eusocial and solitary alleles); a bistable area, where either allele spreads to fixation if common; and a solitary area, where the solitary allele spreads to fixation from any starting frequency. 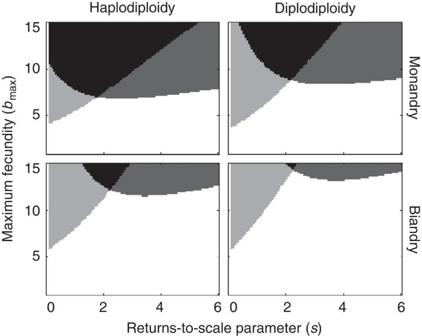Figure 2: Evolution of obligate eusociality based on a dominant allele. In parameter space (bmax;s) of the function mapping fecundity on colony size, there is a eusocial area (black), a bistable area (dark grey), a mixed area (light grey), and a solitary area (white). Settings:N=4;β=0.1;dx=dy=dw=d(n)=0.1. Figure 2: Evolution of obligate eusociality based on a dominant allele. In parameter space ( b max ; s ) of the function mapping fecundity on colony size, there is a eusocial area (black), a bistable area (dark grey), a mixed area (light grey), and a solitary area (white). Settings: N =4; β =0.1; d x = d y = d w = d ( n )=0.1. 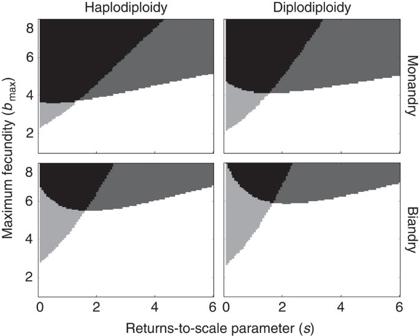Figure 3: Evolution of facultative eusociality based on a dominant allele. In parameter space (bmax;s) of the function mapping fecundity on colony size, there is a eusocial area (black), a bistable area (dark grey), a mixed area (light grey), and a solitary area (white). Settings:N=4;β=0.1;dx=dy=dw=d(n)=0.1. Full size image Figure 3: Evolution of facultative eusociality based on a dominant allele. In parameter space ( b max ; s ) of the function mapping fecundity on colony size, there is a eusocial area (black), a bistable area (dark grey), a mixed area (light grey), and a solitary area (white). Settings: N =4; β =0.1; d x = d y = d w = d ( n )=0.1. 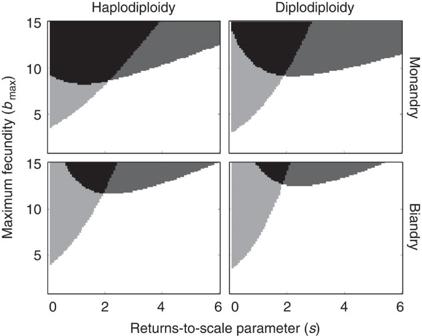Figure 4: Evolution of obligate eusociality based on a recessive allele. In parameter space (bmax;s) of the function mapping fecundity on colony size, there is a eusocial area (black), a bistable area (dark grey), a mixed area (light grey), and a solitary area (white). Settings:N=4;β=0.1;dx=dy=dw=d(n)=0.1. Full size image Figure 4: Evolution of obligate eusociality based on a recessive allele. In parameter space ( b max ; s ) of the function mapping fecundity on colony size, there is a eusocial area (black), a bistable area (dark grey), a mixed area (light grey), and a solitary area (white). Settings: N =4; β =0.1; d x = d y = d w = d ( n )=0.1. 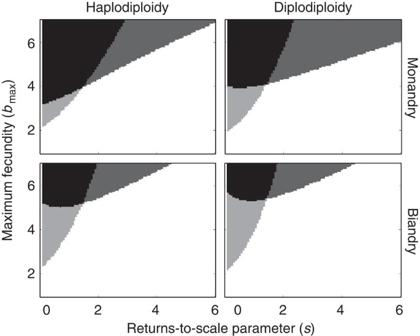Figure 5: Evolution of facultative eusociality based on a recessive allele. In parameter space (bmax;s) of the function mapping fecundity on colony size, there is a eusocial area (black), a bistable area (dark grey), a mixed area (light grey), and a solitary area (white). Settings:N=4;β=0.1;dx=dy=dw=d(n)=0.1. Full size image Figure 5: Evolution of facultative eusociality based on a recessive allele. In parameter space ( b max ; s ) of the function mapping fecundity on colony size, there is a eusocial area (black), a bistable area (dark grey), a mixed area (light grey), and a solitary area (white). Settings: N =4; β =0.1; d x = d y = d w = d ( n )=0.1. Full size image We find that haplodiploidy and monandry, compared with diplodiploidy and biandry, increase the range of conditions under which eusociality can evolve and be stable. This result is robust with respect to assumptions about the eusocial allele's dominance ( Figs 2 and 3 ) or recessiveness ( Figs 4 and 5 ). If workers are permanently sterile (obligate eusociality; Figs 2 and 4 ), eusociality evolves less easily than if workers retain the ability to reproduce in the event of their queen's death (facultative eusociality; Figs 3 and 5 ). This supports the intuitive idea that facultative eusociality is a likely intermediate stage during the evolution of obligate eusociality. Phenotypic associations The extent of positive association between rare phenotypes mediates synergies between such phenotypes, with ramifications for population dynamics and selection. Here we show that, for a given female of a rare phenotype A , the expected proportion of her sisters sharing the same phenotype is larger in a haplodiploid than in a diplodipoid species. Consider a rare allele A for phenotype A in a large population where males and female pair at random. If A is dominant and the population is diplodiploid, daughters with phenotype A will mainly arise from pairings of the genotype combination Aa × aa ; other genotype combinations involving A will be much rarer. Among the daughters derived from such pairings, 50% will have phenotype A (with genotype Aa ). Compare this with a similar situation in a haplodiploid population, where A will arise mainly from pairings of genotype combinations Aa × a and aa × A . A is now present in 50% of daughters from Aa × a pairings and 100% of daughters from aa × A pairings. Thus, for a given daughter of phenotype A , the expected proportion of sisters sharing the same phenotype is larger in a haplodiploid than in a diplodipoid species. If we, instead, consider that A is recessive, then daughters with phenotype A will mainly arise from Aa × Aa pairings in a diplodiploid species, leading to ¼ of daughters with phenotype A . In a haplodiploid species, the relevant genotype combination is Aa × a , leading to 50% of daughters with phenotype A . Again, for a given daughter of phenotype A , the expected proportion of sisters sharing the same phenotype is larger in a haplodiploid than in a diplodipoid species. Superficially, our results appear to support the classic 'haplodiploidy hypothesis', which states that haplodiploid species are pre-disposed for the evolution of eusociality because females in such species are more closely related to their sisters (with a relatedness coefficient r =0.75) than they are to their own offspring ( r =0.5) [13] . Following the recognition that haplodiploidy simultaneously reduces the relatedness between sisters and brothers (to r =0.25) [14] , this hypothesis is no longer considered to be of general importance [5] , [6] , [7] . In our model, however, haplodiploidy favours eusociality for a subtle and previously unrecognized reason. Because haplodiploidy strengthens the extent of positive assortment between phenotypes, it enables synergies between globally rare but locally common phenotypes. For example, in a situation where a queen's reproductive rate b ( n ) is an accelerating function of colony size (so that small colonies are relatively inefficient compared with larger colonies; s >1 in Fig. 1 ), the direction of selection on the eusocial allele depends on the time that its carriers typically spend in smaller or larger colonies. With strong positive assortment between initially rare cooperators, colonies can reach an efficient size more quickly, which greatly facilitates the evolution of eusociality. Haplodiploidy can also make established eusociality more stable against the invasion of rare solitary alleles ( Figs 2 and 3 , although this effect is less robust Figs 4 and 5 ). Again, this is because haplodiploidy strengthens the positive assortment between rare phenotypes, which penalizes 'free-riders' who thrive best when surrounded by 'cooperators', rather than by their own kind. Solitary alleles can be considered 'free-riders' in this context because a solitary allele, if present among the parental genotypes that constitute the genetic makeup of a colony, does not contribute to worker production (that is, it does not cause offspring to become workers) while benefiting from the local work force and being overrepresented in dispersing offspring. Given the recent debate about the merits of kin selection [10] , [15] , [16] , [17] , [18] , [19] , [20] , [21] , it is worth emphasizing that models that are not explicitly phrased in terms of 'inclusive fitness', including ours, nevertheless allow kin selection to operate. Social interactions between relatives have a crucial role for the total selection experienced by an allele. It has been pointed out that kin structure is one of multiple ways to create positive assortment between cooperators [22] , [23] . Like haplodiploidy, monandry positively assorts cooperative phenotypes (via kinship), thus strengthening the synergies described above. Although our model highlights the importance of demography, this does not come at the expense of the general usefulness of simple rules (for example, Hamilton's) when deriving empirically testable predictions in the field of social evolution [24] . Indeed, our model is in line with such work, producing simple predictions such as support for the hypothesis [12] , [25] that eusociality can evolve more easily in species with monandrous females. Comparative evidence suggests that all known clades of eusocial hymenopteran insects evolved from monandrous ancestors, even though several of them later evolved polyandry [9] . A negative relationship between promiscuity and the evolution of cooperative breeding in birds [8] likewise supports a role of monogamy in favouring the evolution of helping behaviour, although no birds are classified as eusocial. The present work strengthens the theoretical foundation of these empirical results, which has recently been questioned based on an individual-based simulation model that has compared invasion speed of a social allele under monandry versus biandry, instead of comparing the parameter space where evolution of sociality is predicted or not [17] . Our model also shows that the logical difficulties that have plagued the haplodiploidy hypothesis [5] , [6] , [7] can be overcome once the ecology of cooperation (in terms of 'returns to scale') is taken into account by explicitly following the demographic and genetic changes in growing colonies. Together, haplodiploidy and monogamy are a stronger force promoting eusociality than monogamy alone. This reinstates the long-suspected association between the unusual genetic system of the Hymenoptera and eusociality. A role of synergy in kin selection has been recognized before [22] , [26] , [27] , [28] , but its interaction with demographic and genetic processes that assort cooperators together has not been fully recognized. Synergy arises when joint efforts achieve more than the sum of their parts. For example, two independently working foragers that contribute to a common pool of resources in a stochastic environment will disproportionally reduce the likelihood of colony-level resource shortage compared with one, even if their foraging tactics are identical. Moreover, in eusocial insects, synergy often relies on division of labour, which may increase s and b max greatly. With certain pre-adaptations in place (for which there is evidence in the Hymenoptera [29] , [30] , [31] ), division of labour may emerge as a direct consequence of offsprings' failure to disperse [32] , which according to our model feeds back to enhance the evolution of eusociality. To achieve strong phenotypic effects with synergy, a single locus does not have to bring about much else than a failure to disperse; a worker will simply perform similar parenting duties as a nest foundress would have done after egg-laying. This justifies our assumption that a single locus can have a strong phenotypic effect. Indirect evidence for increasing returns to scale, at least for small colony sizes, can also be found in the observation that colony sizes in nature are typically ≫ 1. We encourage explicit studies of colony economics to yield direct estimates of s (or similar relevant parameters in tailor-made models for particular types of colony demography), while also noting that future studies could highlight more flexible shapes of returns to scale, and the associated dispersal rules. Thus, while our model is deliberately kept simple to illustrate principles of general importance, more complex scenarios (including gradual cumulative adaptation at multiple loci, and co-evolutionary feedbacks between variables such as N , b max , s ) present exciting avenues of further work. In view of recent suggestions that high within-colony relatedness may be a mere consequence of eusociality, without having a causal role in its evolution [10] , [11] , our results firmly show that the relatedness structure of a population can be of decisive importance for whether the transition to eusociality occurs. Simultaneously, this transition becomes more likely when assortment between cooperator genotypes is strengthened via haplodiploidy, and when the benefits of cooperation are enhanced in larger colonies (ecological efficiency). A proper understanding of the evolution of eusociality requires the simultaneous consideration of mating system, genetic system, and ecology. Model For a given genetic system and mating system, we identify K possible colony types that differ with respect to the genotype combinations of the founding individuals ( Supplementary Tables 1–4 ; for an overview of the variables used, see Supplementary Table S5 ). Colony size n ranges from n =1 (a reproductive female with no workers) to a maximum of n=N (a reproductive female with N −1 workers). Denoting A and a as the eusocial and the solitary allele, respectively, we let q π, n be the probability that a female offspring of genotype π , produced in a colony of size n , develops a worker phenotype. For colony sizes satisfying n < N , we let q AA, n =1; q Aa, n =1; q aa, n =0 if A is dominant, and q AA, n =1; q Aa, n =0; q aa, n =0 if A is recessive. Because we assume that all offspring produced in colonies of size N disperse and thus never become workers, we have q π, N =0 for any genotype π . We consider a large population whose total size we express as , where x is the number of virgin females, y is the number of males, and X k,n is the number of colonies of type k and size n . Reproductive females reproduce at rate φb ( n ), where examples of b ( n ) are shown in Figure 1 and the coefficient φ =1/(1+ ω ) implements density-dependence to ensure that the population converges to a stable size. The number of virgin females of genotype π in the mating pool changes over time as where the expression in large brackets sums the production of dispersing daughters across colonies of all types and sizes. Here, υ π,k is the probability that a given daughter produced in a type k colony is of genotype π (see Supplementary Tables 1–4 ). The expression x π ( βy + d x ) in equation (1) accounts for females that disappear from the mating pool owing to mating (this happens at a rate proportional to y, the number of males in the mating pool, scaled by parameter β ) or due to death (at rate d x ). To focus on the effect of shared paternity, we assume that mating takes the same amount of time regardless of whether a female mates once or twice. This is a reasonable assumption if males are numerous and/or occur in the habitat in a clumped fashion, so that a female that finds one male will usually find a second male close by. The summand θ in equation (1) represents any workers that join the mating pool after their queen's death. If workers are permanently sterile (the obligate eusociality case), θ =0. If workers retain the capacity to reproduce (the facultative eusociality case), where d ( n ) is the death rate of queens in size n colonies, ( n –1) is the number of workers dispersing in the event of their queen's death, and is the proportion of workers with genotype π in a type k colony. Here, i is an index running over all possible genotypes and n can take any value satisfying n < N . The number y π of males of genotype π changes over time as where the expression in brackets sums the production of sons across colonies of all types and sizes, and d y is the male mortality rate. The probability that a daughter produced in a type k colony of size n (satisfying n < N ) becomes a worker is given by . The number of type k colonies of size 1 changes over time as where χ k is the rate at which type k colonies are founded when males and virgin females of the appropriate genotypes mate (see Supplementary Tables 1–4 ), d w is the rate at which workers die (making size 2 colonies shrink to size 1), d (1) is the rate at which queens in size 1 colonies die, and φb (1) w k,1 is the rate at which size 1 colonies grow to size 2 due to a worker being produced. The quantity of type k colonies of size n (where 1< n < N ) changes over time as where X k,n −1 φb ( n −1) w k is the rate at which size n colonies arise due to worker production in size n −1 colonies, d w nX k,n +1 is the rate at which size n colonies arise by the death of one of the n workers in a n +1 size colony, d ( n ) is the rate at which queens in size n colonies die, and φb ( n ) w k is the rate at which size n colonies grow to size n +1 due to a worker being produced. The quantity of type k colonies of size N changes over time as where X k ,N −1 φb ( N −1) w k is the rate at which size N colonies arise due to worker production in size N –1 colonies, and X k ,N d ( N ) is the rate at which queens in size N colonies die. We studied the dynamics of this system using the Euler approximation [33] , with A =0.01 and A =0.99 as the starting frequencies of the eusocial allele, considering asymptotic change rather than initial transient dynamics. How to cite this article: Fromhage, L. & Kokko, H. Monogamy and haplodiploidy act in synergy to promote the evolution of eusociality. Nat. Commun. 2:397 doi: 10.1038/ncomms1410 (2011).